Mutational landscape of gingivo-buccal oral squamous cell carcinoma reveals new recurrently-mutated genes and molecular subgroups Gingivo-buccal oral squamous cell carcinoma (OSCC-GB), an anatomical and clinical subtype of head and neck squamous cell carcinoma (HNSCC), is prevalent in regions where tobacco-chewing is common. Exome sequencing ( n =50) and recurrence testing ( n =60) reveals that some significantly and frequently altered genes are specific to OSCC-GB ( USP9X , MLL4 , ARID2 , UNC13C and TRPM3 ), while some others are shared with HNSCC (for example, TP53 , FAT1 , CASP8 , HRAS and NOTCH1 ). We also find new genes with recurrent amplifications (for example, DROSHA , YAP1 ) or homozygous deletions (for example, DDX3X ) in OSCC-GB. We find a high proportion of C>G transversions among tobacco users with high numbers of mutations. Many pathways that are enriched for genomic alterations are specific to OSCC-GB. Our work reveals molecular subtypes with distinctive mutational profiles such as patients predominantly harbouring mutations in CASP8 with or without mutations in FAT1. Mean duration of disease-free survival is significantly elevated in some molecular subgroups. These findings open new avenues for biological characterization and exploration of therapies. Oral squamous cell carcinoma (OSCC) is the eighth most common cancer worldwide [1] and is the leading cancer among men in India [2] . Annually >260,000 new cases arise and ~128,000 deaths occur [3] . Tobacco smokers have 27 times higher rate of oral cancer than non-smokers [4] . Chewing betel-quid comprising betel leaf ( Piper betle ), areca nut ( Areca catechu ) and slaked lime (predominantly calcium hydroxide), with or without tobacco, is traditional and popular in India and is known to cause oral cancer [5] . Widespread use of smokeless tobacco in India, which explains over half of the oral cancers [6] , is common among the youth (13–15 years): 14.1% among boys and 6% among girls [7] . Human papilloma virus (HPV) infection is an established risk factor, with prevalence in OSCC ranging between 20 and 50% across geographical regions [8] . Oral cancer predominantly presents as tongue cancer (~65%) in the West, while in India it predominantly (~60%) affects the gingivo-buccal region, comprising buccal mucosa, retro-molar trigone and lower gum [9] , [10] . Patients with oral squamous cell carcinoma of the gingivo-buccal region (OSCC-GB) mostly present at advanced stages (stages III and IV) and have a very high loco-regional failure rate and mortality despite best multimodal treatment [11] . The two earlier exome-sequencing studies [12] , [13] on head and neck squamous cell carcinoma (HNSCC), included patients affected at a heterogeneous set of anatomical sites, including the oral cavity. Both studies identified TP53 , CDKN2A , PIK3CA , HRAS and NOTCH1 to be frequently mutated. A recent integrative genomic analysis of OSCC [14] additionally discovered frequent mutation of CASP8 defining a new molecular subtype, and identified four major driver pathways—mitogenic signalling, Notch, cell cycle and TP53. Another recent study [15] has identified that the tumour suppressors CTNNA2 and CTNNA3 are frequency mutated in laryngeal carcinomas. Oral cavity comprises sub-sites with distinct biological features [16] . It is therefore likely that genes driving cancers in these sub-sites may be different. Here we characterize the somatic mutation landscape of OSCC-GB, the most common and anatomically homogeneous cancer in India that constitutes a significant global cancer burden. We identify the nature and extent of genomic alterations specific to this anatomical subset (OSCC-GB) within the wider anatomical set (HNSCC) and study their prognostic implications. Our study reveals new genes and mutationally enriched pathways that are specific to OSCC-GB, and suggest molecular subtypes that may be associated with significantly better disease-free survival (DFS) period. Patient description With informed consent, blood and tumour tissues were collected at the time of surgical excision, from 50 treatment-naive OSCC-GB patients (discovery set) who underwent a comprehensive staging, curative resection, post-operative radiotherapy±chemotherapy and follow-up at ACTREC. Only patients with concordant histologic diagnosis by two independent reviewers were included. Sections of tumours that contained at least 80% tumour nuclei among total cellular nuclei were used for DNA isolation and quantitation (Methods). Data on demography, risk factors, clinical, radiological and histopathological features, treatment parameters and disease status at follow-up were collected. Each patient was followed up until death or recurrence. Summary statistics are provided in Supplementary Table S1 . Most (88%) patients were male, ~50% were between 40 and 50 years of age, 96% were exposed to tobacco±alcohol and 94% presented at advanced stage III/IV. Surgical dissection and histological examination of regional nodes confirmed nodal metastasis in 50% cases. Infection with HPV and Herpes Simplex Virus (HSV) was detected in 26% (all infected with high-risk subtypes; 22% with subtype 16, 2% with subtype 18 and 2% with mixed subtypes) and 2% of patients, respectively. In addition, 60 independent OSCC-GB patients (confirmation set) were similarly recruited and biospecimens collected from them were similarly analysed for confirmation of genomic discoveries. Characteristics of patients who comprised the ‘confirmation set’ were similar to those of the ‘discovery set’: mean ages (in years) of patients in discovery and confirmation sets were 48.0 and 47.5, respectively ( t -test P -value for equality of means >0.05) and, gender proportions were not different ( Z -test P -value for equality of proportions >0.05). However, the proportion of HPV-positive patients in the confirmation set was lower, resulting in an overall proportion of 19.3%. Exome sequencing and verification Coding exons of 19,806 protein coding genes and 1,040 non-coding RNAs were sequenced from DNA isolated from blood (to exclude inherited sequence variants) and primary tumour of each patient. Of these, coding exons of 15,906 genes and 394 non-coding RNAs were sequenced independently on two orthogonal sequencing platforms (Illumina HiSeq 2000 and Roche GS-FLX). Because of the double-platform sequencing and verification strategy used, our data are of very high quality. Mean±s.d. depths of sequencing for blood and tumour DNA on HiSeq 2000 were 37.58±6.76 and 36.67±8.44, respectively; the corresponding estimates for GS-FLX were 24.92±2.52 and 35.43±5.73, respectively. Details for each patient are provided in ( Supplementary Table S2 ). Concordance of germline single-nucleotide variant (SNV) genotype calls on the two sequencing platforms was 92.36%. Concordance estimate of germline genotypes for ~10,000 SNVs that were also present on the Illumina Omni Quad DNA microarray was in excess of 99.5% for each deep-sequencing platform. Of all SNVs in the genes that were frequently and significantly mutated and could be sequenced only on one platform, 98% were verified using Ion Torrent PGM (Life Technologies) at a mean depth of 200 × . Since TP53 is the most frequently mutated HNSCC gene, we Sanger-sequenced TP53 . Somatic mutations in TP53 in seven patients that were detected by Sanger sequencing were unreported in massively parallel sequencing data because of the lack of adequate coverage, even though reads with the relevant mutant allele were present in the data on each of these seven patients. All TP53 mutations detected by massively parallel or Sanger sequencing were catalogued. Copy number variations (CNVs) were identified by analysing genotype data generated using DNA microarrays; most were verified by real-time PCR. Mutational landscape of OSCC-GB Coding regions of genomes of the 50 patients contained 5,646 somatic variants, of which 176 (3%) were indels and the remaining were single-nucleotide substitutions. Of the single-nucleotide substitutions, 1,398 (24.8%) were predicted to be synonymous; 3,629 (64.3%), missense; 311 (5.5%), nonsense and 104 (1.8%), splice site. Among the indels, frameshift deletions were the most common (56.2%). The mean numbers of variants (single-nucleotide variants (SNVs) and indels) per patient, including and excluding synonymous variants, were 113 (range: 13–939) and 85 (range: 12–637), respectively. The sequencing depth for the patient with the lowest number of verified variants averaged over the two platforms and the two DNA sources was 36.98±6.69. Average mutation rates per Mb, including and excluding synonymous mutations, were estimated to be 3.52±0.59 and 2.65±0.41, respectively ( Supplementary Table S3 ). The mean number of variants (range: 1–39) in non-coding RNA genes per patient was 7.56±5.99 ( Supplementary Data 1 and Supplementary Table S4 ). Primary tumours of 13 (26%) patients carried high-risk (16 and/or 18) HPV subtypes. Contrary to an earlier report [12] on HNSCC, in the OSCC-GB patients we did not find a statistically significant difference ( Z -test P -value for equality of proportions >0.05) in the proportions of different types of mutations in patients with or without HPV infection, and found that a high proportion (61%) of HPV-associated tumours carried TP53 mutations ( Fig. 1 ). Similarly, contrary to an earlier report [13] , the HPV-infected patients did not exhibit a lower mutation rate (4.07 mutations per Mb) compared with HPV-negative patients (3.36 mutations per Mb). 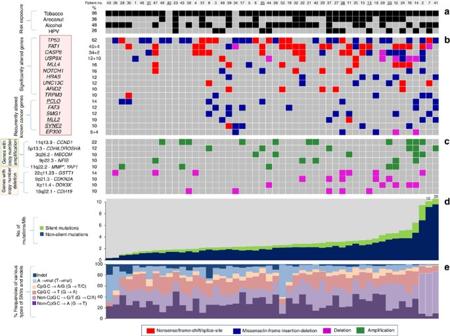Figure 1: Data summary of 50 gingivo-buccal oral cancer patients. Demographic characteristics, environmental exposures and landscape of genomic alterations are shown. These data have been organized in increasing order of the total number of mutations observed in each patient. Patient numbers that are underlined are female; the remaining are male. (a) Exposures to known risk factors, including HPV. Tobacco exposure includes all forms of tobacco use. Exposed patients are indicated as a filled square. (b) Ten genes found to be significantly altered, indicated in bold, are arranged in descending order of the percentage of patients who showed alterations (SNV and CNV, which are indicated with a ‘+’ separator). Types of alterations are colour-coded; the colour-coding scheme is indicated at the bottom of the figure. Six genes that were previously identified to be frequently altered in other cancers and were found to be present in at least 10% of the patients included in this study are also listed. Three genes that were found to be frequently mutated in an earlier study on head and neck squamous cell carcinoma13are underlined. (c) Genes of relevance that are amplified (5 genes) or deleted (4 genes) in at least 10% of patients (note: CNVs detected in genes such as olfactory receptor genes are not listed because of lack of evidence of their involvement in cancers). All amplifications are full-gene amplifications; the deletion involvingGSTT1is a full-gene deletion, while the others are partial deletions. (d) Numbers of silent and non-silent mutations per Mb (note: for patient nos. 7 and 41, the total number of mutations per Mb, 12 and 29, respectively, exceeds the scale; hence, these numbers are displayed). (e) Spectrum of mutations for each patient: percent frequencies of various categories of SNVs and indels. The bars representing the frequency of C>G/T at non-CpG sites are highlighted for the three patients 2, 7 and 41 (see text for explanation), *Entire MMP gene-family on chromosome 11 was amplified. Figure 1: Data summary of 50 gingivo-buccal oral cancer patients. Demographic characteristics, environmental exposures and landscape of genomic alterations are shown. These data have been organized in increasing order of the total number of mutations observed in each patient. Patient numbers that are underlined are female; the remaining are male. ( a ) Exposures to known risk factors, including HPV. Tobacco exposure includes all forms of tobacco use. Exposed patients are indicated as a filled square. ( b ) Ten genes found to be significantly altered, indicated in bold, are arranged in descending order of the percentage of patients who showed alterations (SNV and CNV, which are indicated with a ‘+’ separator). Types of alterations are colour-coded; the colour-coding scheme is indicated at the bottom of the figure. Six genes that were previously identified to be frequently altered in other cancers and were found to be present in at least 10% of the patients included in this study are also listed. Three genes that were found to be frequently mutated in an earlier study on head and neck squamous cell carcinoma [13] are underlined. ( c ) Genes of relevance that are amplified (5 genes) or deleted (4 genes) in at least 10% of patients (note: CNVs detected in genes such as olfactory receptor genes are not listed because of lack of evidence of their involvement in cancers). All amplifications are full-gene amplifications; the deletion involving GSTT1 is a full-gene deletion, while the others are partial deletions. ( d ) Numbers of silent and non-silent mutations per Mb (note: for patient nos. 7 and 41, the total number of mutations per Mb, 12 and 29, respectively, exceeds the scale; hence, these numbers are displayed). ( e ) Spectrum of mutations for each patient: percent frequencies of various categories of SNVs and indels. The bars representing the frequency of C>G/T at non-CpG sites are highlighted for the three patients 2, 7 and 41 (see text for explanation), *Entire MMP gene-family on chromosome 11 was amplified. Full size image Nearly all (96%) of the OSCC-GB patients included in this study were exposed to tobacco (chewing±smoking). The C:G>A:T transversion, a preponderance of which is a feature of mutations induced by tobacco carcinogens [17] , was found in high proportion (61%) in the OSCC-GB tumours; much higher than observed (15–26%) in various cancers not associated with tobacco [18] , and also in the general population (31%) ( Supplementary Fig. S1 ). We observed ( Supplementary Fig. S2 ) that C:G>A:T transversion (tobacco signature) occurred at 5′-GCX (C is the mutated base, and X is any base) at frequencies significantly ( Z -test P -values for equality of proportions ranged between 3.8 × 10 −12 and 0.02) higher than expected. There was an over-representation of C>T and C>G mutations at 5′-TCX ( Z -test P -values for equality of proportions ranged between 4.1 × 10 −130 and 1.4 × 10 −14 ), similar to findings on breast cancer [19] and C>T somatic mutations were predominant at non-CpG sites ( Fig. 1e ), contrary to what is normally observed in the germline ( Supplementary Fig. S2D ). Interestingly, three OSCC-GB patients (patient nos 2, 7 and 41; Fig. 1 ), all tobacco users, who harboured large numbers of mutations (315, 391 and 939, respectively), had relatively smaller proportions of C:G>A:T transversion, compared with the C:G>G:C transversion, which was the highest proportion in all the three patients ( Fig. 1e ). C>G transversion is caused by 8-oxoguanine [20] , a DNA lesion formed by exposures to tobacco and reactive oxygen species [21] . Over activity of APOBEC family of genes has been reported to result in C>T and C>G mutations at TpCpX trinucleotides in diverse human cancers [22] . Five new genes associated with OSCC-GB Somatic mutations were observed in 4,109 genes; 981 were mutated in ≥2 tumours ( Supplementary Data 1 ), of which 45 were mutated in ≥10% of the tumours. Among these 45 genes, those that were mutated at a significantly higher than the background rate (ascertained using data on only SNVs and indels, but not CNVs, in the gene), after appropriately adjusting for their lengths and base compositions, using the MuSiC algorithm [23] , and independently verified by the MutSigCV algorithm [24] , were considered as genes associated with OSCC-GB. Ten genes were significantly mutated (all FDR-corrected P -values using only the SNV data, but not the CNV data, were <0.05) and altered: TP53 (0.62+0=0.62; that is, 62% of patients with SNVs and 0% with CNVs), FAT1 (0.40+0.04=0.44), CASP8 (0.34+0.02=0.36), USP9X (0.12+0.10=0.22), MLL4 (0.16+0=0.16), NOTCH1 (0.16+0=0.16), HRAS (0.12+0=0.12), UNC13C (0.12+0=0.12), ARID2 (0.10+0=0.10) and TRPM3 (0.10+0=0.10). Some of these genes— TP53 , FAT1 , CASP8 , HRAS and NOTCH1 —were previously implicated in HNSCC [12] , [13] , [25] . Mutations, many truncating, in FAT1 occurred at a higher frequency than reported earlier [13] (12%). Two other members of the FAT family, FAT3 and FAT4 , were also mutated in 12 and 8% of OSCC-GB patients, respectively. We have found five new genes associated with OSCC-GB— USP9X , MLL4 , ARID2 , UNC13C and TRPM3 —that are frequently altered (10–22% of patients) at a rate significantly higher than the background rate, ascertained by GenomeMuSiC [23] , with two of the three FDR-corrected P -values of Z -test for testing equality of proportions being <0.2 and independently verified as statistically significant ( Z -test P -value for equality of proportions <0.05) by MutSigCV [24] ( Supplementary Table S5 ). USP9X encodes a deubiquitinating enzyme [26] and is a tumour suppressor [27] ; 22% of OSCC-GB patients harboured DNA alterations (mutations and CNVs) in USP9X . We have found copy number loss and truncating mutations in USP9X ( Fig. 1 ), consistent with its role as a tumour suppressor [27] . Two chromatin remodelling genes, MLL4 and ARID2 were also significantly mutated ( Fig. 1 ), primarily with truncating mutations. MLL4 acts as a co-activator of the tumour suppressor p53 and regulates trimethylation of H3K4 (refs 28 , 29 ). ARID2 encodes a protein that is involved in transcriptional activation and repression of genes by chromatin remodelling [30] , [31] . The remaining two new genes associated with OSCC-GB that were identified in this study— UNC13C and TRPM3 —belong to neurotransmitter release-related processes [32] , [33] . TRPM3 is a potential tumour suppressor that possibly acts synergistically with miR-204 (ref. 34 ). Two or more mutations in the same patient were observed ( Supplementary Table S6 ) in: TP53 (4/31; that is, 4 patients harboured ≥2 mutations in TP53 among the 31 patients who harboured mutations in this gene), FAT1 (3/20), MLL4 (2/8) and NOTCH1 (1/8). Observed mutations in only TP53 were clustered; the clustering was in the DNA-binding domain ( Supplementary Fig. S3 ). Of the eight known [35] somatically mutated hotspots in cancer, only four were mutated in multiple OSCC-GB patients ( Supplementary Table S7 ). Several cancer-associated genes were frequently, but not significantly, mutated in OSCC-GB. These include SYNE2 (10%) and SYNE1 (6%), consistent with a previous HNSCC study [13] , involved in nuclear polarity and spindle orientation that function upstream of NOTCH1 signalling in the squamous cell differentiation pathway [36] . PCLO , a gene involved in calcium signalling, was mutated in 14% of OSCC-GB patients; this frequency is similar (12%) to a previous report on HNSCC [13] , although a recent study [24] has claimed that PCLO is not a cancer gene. SMG1 , mutated in 12% of patients, acts as a genotoxic stress-activated protein kinase that can phosphorylate p53 and is required for optimal p53 activation after cellular exposure to genotoxic stress [37] . The well-known tumour suppressor, MLL2 , was mutated in 10% of the OSCC-GB patients. There is also a long tail of mutations in known cancer genes that were mutated in <10% of OSCC-GB patients ( Supplementary Fig. S4 ). Recurrence testing in independent samples Targeted massively parallel resequencing of the 10 significantly mutated genes (SMGs) in 60 independent OSCC-GB tumour/normal pairs showed that all the genes were mutated in 5–72% of the tumours and that FAT1 was significantly ( Z -test P -value for equality of proportions=0.01) less frequently mutated (18% of patients in confirmation set versus 40% in the discovery set). This lower frequency was partially compensated by a higher (72 versus 62%; Z -test P -value for equality of proportions=0.28) frequency of mutated TP53 . In the discovery and confirmation sets, the frequencies with which the five new OSCC-GB genes were mutated were similar ( Supplementary Table S8 ). Copy number variations Genomic segments with more than three copies or loss of at least one copy in ≥10% of patients were identified ( Supplementary Data 2 ). CNVs were also identified in genes with recurrent mutations (SNVs and/or indels) in OSCC-GB patients. We found and confirmed ( Supplementary Table S9 ) several genes, not previously reported to carry CNVs in HNSCC, with recurrent amplification, such as DROSHA (12% of patients), MECOM (10%), MMP gene cluster region on chromosome 11q that includes YAP1 (10%); NFIB (10%); or with recurrent homozygous deletion, such as DDX3X (10%). Among those genes reported earlier in HNSCC, we found amplifications of CCND1 (22%) and TP63 (8%), homozygous deletion of GSTT1 (14%) and heterozygous deletions of CDKN2A [25] (10%) and CDH19 (10%). TP63 gene product is abundant in squamous epithelia; this protein promotes renewal of basal keratinocytes by a mechanism that requires downregulation of NOTCH1 and CDKN2A [13] . Both NOTCH1 and CDKN2A were frequently mutated in OSCC-GB. The gene encoding cell cycle protein D1 ( CCND1 ) was earlier reported to be amplified in ~30% of HNSCC patients [38] ; observed frequency of amplification in OSCC-GB was 22%, mostly (81%) in HPV-negative tumours consistent with an earlier report [25] . Deletions in CSMD1 , a putative tumour suppressor implicated in diverse cancers including HNSCC [39] , [40] , were found in a substantial fraction (26%) of OSCC-GB patients. Pathway analysis Alterations in genes that were frequently and significantly mutated among OSCC-GB patients were considered as the drivers of pathways for initiation and progression. SNV and Indel data analysed with PathScan module in GenomeMuSiC [23] identified 16 statistically significant KEGG pathways based on enrichment of mutations ( Table 1 ). CNV data were added to identify additional drivers in enriched pathways. Many important regulatory pathways not earlier reported to be associated with HNSCC or oral cancer were enriched in OSCC-GB patients. Enrichment was assessed by likelihood-ratio test for an increase in the overall mutation rate adjusted for lengths of genes in a pathway and for clustering of mutations. These are, neurotrophin signalling ( P =7.1 × 10 −6 ), Wnt signalling ( P =9.0 × 10 −4 ), dorso-ventral axis formation ( P =2.4 × 10 −3 ) and axon guidance ( P =3.9 × 10 −3 ). Table 1 Significantly altered pathways in gingivo-buccal oral squamous cell carcinoma. Full size table We also identified several pathways that are known to be important for cancer and HNSCC pathogenesis: p53 signalling ( P =4.87 × 10 −9 ), apoptosis ( P = 5.21 × 10 −9 ), PI3K–Akt signalling ( P =1.0 × 10 −3 ) and Notch signalling ( P =4.4 × 10 −2 ). Some other pathways that are not known to be associated with cancer were significantly altered in OSCC-GB patients; these include neuroactive ligand–receptor interaction ( P =0.026), serotonergic synapse ( P =0.046). We note that enrichment of the chromatin remodelling pathway in OSCC-GB could not be detected because the KEGG database does not contain information on many known chromatin remodelling genes. Molecular subgroups and disease-free survival Since the characteristics and genomic profiles of patients belonging to the discovery and confirmation sets were similar, we pooled data of all patients ( n =50+60=110) to identify possible existence of molecular subgroups in OSCC-GB. Numbers of alterations (SNVs or indels) in the SMGs in each OSCC-GB patient were used in this analysis. Squared Euclidean distance was used to measure dissimilarity of mutational profiles between patients. Ward’s [41] method was used for agglomerative clustering. Three broad clusters were identified ( Fig. 2 ). CASP8 is mutated, predominantly (54.3%) with truncating mutations, in 35 (92.1%) of the 38 patients belonging to first cluster (C 1 ). In addition to CASP8 , 21 (60%) of these 35 patients also possessed mutations (predominantly truncating) in FAT1 and/or NOTCH1 ( Fig. 2 ). TP53 is mutated in all of the 43 patients who belong to the second cluster (C 2 ), predominantly with missense and in-frame indels (67.4%). The third cluster (C 3 ) comprising 29 patients carry alterations in a heterogeneous set of genes, although a high proportion (55%) of them carries mutations in MLL4 and USP9X . Patients with mutations in these two genes are essentially restricted to the third cluster. Each broad cluster comprises mutationally more homogeneous subclusters ( Fig. 2 ). 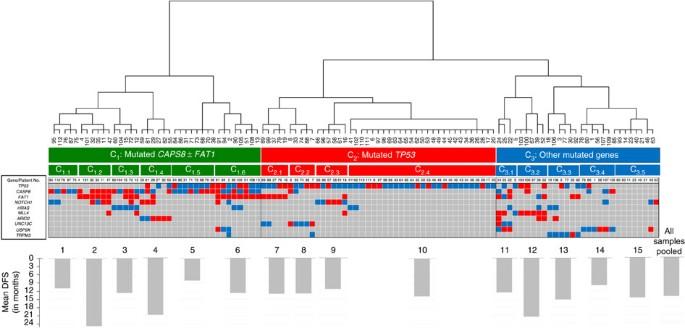Figure 2: Clustering of gingivo-buccal oral cancer patients based on mutational profiles. Hierarchical clustering of 110 gingivo-buccal oral squamous cell carcinoma patients based on 10 significantly and frequently mutated genes form three broad clusters (C1–C3) with the following essential characteristics: (a) Patients with mutations inCASP8with or without mutations inFAT1, (b) patients with mutations inTP53and (c) patients with mutations in various other genes. Within each cluster, there are multiple subclusters. The duration (in months) of disease-free survival averaged over patients belonging to each subcluster is provided in the panel below. The mean duration of disease-free survival is long for three subclusters comprising patients with mutations in (i)CASP8,NOTCH1andFAT1(C1.2), (ii)CASP8,NOTCH1andARID2(C1.4) and (iii)MLL4with other genes (C3.2). Filled boxes indicate DNA alterations; red and blue boxes indicate, respectively, nonsense/frame-shift/splice-site and missense/in-frame insertion-deletion. Figure 2: Clustering of gingivo-buccal oral cancer patients based on mutational profiles. Hierarchical clustering of 110 gingivo-buccal oral squamous cell carcinoma patients based on 10 significantly and frequently mutated genes form three broad clusters (C 1 –C 3 ) with the following essential characteristics: ( a ) Patients with mutations in CASP8 with or without mutations in FAT1 , ( b ) patients with mutations in TP53 and ( c ) patients with mutations in various other genes. Within each cluster, there are multiple subclusters. The duration (in months) of disease-free survival averaged over patients belonging to each subcluster is provided in the panel below. The mean duration of disease-free survival is long for three subclusters comprising patients with mutations in (i) CASP8 , NOTCH1 and FAT1 (C 1.2 ), (ii) CASP8 , NOTCH1 and ARID2 (C 1.4 ) and (iii) MLL4 with other genes (C 3.2 ). Filled boxes indicate DNA alterations; red and blue boxes indicate, respectively, nonsense/frame-shift/splice-site and missense/in-frame insertion-deletion. Full size image Each patient was followed up after surgery until death or recurrence. The duration of DFS varied from 1 to 39 months, with an overall mean of 14.22±0.93 months. Mean values of DFS duration among subclusters were variable ( Fig. 2 ). For patients belonging to the subclusters C 1.2 (with mutations in CASP8 , NOTCH1 and FAT1 ), C 1.4 (with mutations in CASP8 , NOTCH1 and ARID2 ) and C 3.2 (with mutations in MLL4 and other genes), each comprising six patients (totalling 16% of all patients), the mean DFS duration was significantly longer than the overall mean ( t -test P -values for equality of means were, respectively, 0.01, 0.04 and 0.03). Mean DFS duration of patients belonging to other subclusters did not differ significantly ( t -test P -value for equality of means >0.05) from the overall mean. Among possible predictors of DFS—age at first presentation, tumour stage and regional node involvement (no patient had distant metastasis at first presentation)—only node involvement was statistically significant ( t -test P -value of regression intercept=0.002). The proportion of patients with regional node involvement among those belonging to the subclusters C 1.2 , C 1.4 and C 3.2 (5 of 18 patients) was not significantly different ( P -value of Fisher’s exact two-tailed test=0.073) from that among all patients (59 of 110 patients). For each gene significantly associated with OSCC-GB, we tested whether patients with or without mutations in the gene have altered mean durations of DFS. Except for MLL4 , no such alteration was found for any gene. Patients with mutations in MLL4 ( n =11) had a significantly ( t -test P -value for equality of means=0.047) elevated duration of DFS (20.4±3.1 months) compared with those ( n =99) who did not possess mutations (13.5±0.9 months). Patients who harboured mutations in MLL4 did not exhibit regional node involvement (8 of 11 patients) compared with the pooled set of patients ( P -value of Fisher’s exact two-tailed test=0.12). The Kaplan–Meier survival probability distributions are given in Fig. 3 . 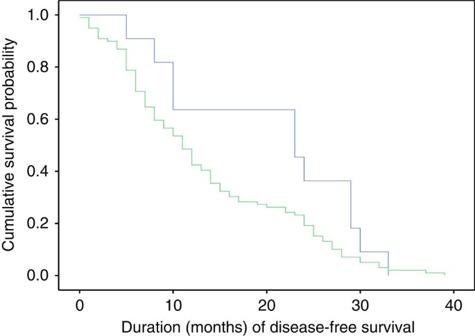Figure 3: Kaplan–Meier probability distributions of disease-free survival. Results are shown for gingivo-buccal oral squamous cell carcinoma patients with (n=11; blue line) and without (n=99; green line) mutations inMLL4. Figure 3: Kaplan–Meier probability distributions of disease-free survival. Results are shown for gingivo-buccal oral squamous cell carcinoma patients with ( n =11; blue line) and without ( n =99; green line) mutations in MLL4. Full size image The high-confidence catalogue of somatic mutations created by massively parallel sequencing on two orthogonal platforms of the exomes of 50 Indian oral squamous cell carcinoma patients with involvement of only the gingivo-buccal complex has revealed many specific features that are different from earlier exome-sequencing studies [12] , [13] , [14] on HNSCC. Mutational profiles of HPV-associated (19.3% in the pooled discovery and confirmation sets of samples, higher than 12–14% found in previous HNSCC studies [12] , [13] ) and HPV-negative OSCC-GB tumours were similar. TP53 mutations occurred on both HPV-positive and -negative backgrounds in nearly equal proportions (~65%; n =110), unlike in the anatomically less homogeneous HNSCC [12] , [13] . Thus, the association between TP53 mutation background and HPV positivity may differ among anatomical sites in HNSCC. Most (96%) of the OSCC-GB patients were exposed to tobacco; hence, the mutational profile of a large fraction (61%) of patients showed a preponderance of C:G>A:T transversions (tobacco signature), which occurred predominantly at 5′-GCX sites. There was also an over-representation of C>T and C>G mutations at 5′-TCX ( P -values ranging from 4.1 × 10 −130 to 1.4 × 10 −14 ), similar to findings in breast cancer [19] . Tobacco users with high numbers of mutations had a relatively smaller proportion of C:G>A:T transversion, compared with the C:G>G:C transversion. The C>G transversion is possibly caused by 8-oxoguanine lesions in the DNA formed by tobacco and reactive oxygen species [20] and/or over activity of APOBEC family of cytidine deaminases together with uracil-DNA glycosylase that generates both C>T transition and C>G transversion at TpCpX trinuclotides [22] . As anatomically HNSCC is a superset of OSCC-GB, many HNSCC driver mutations [12] , [13] were also identified and confirmed as OSCC-GB drivers. However, the frequencies with which these genes were mutated among OSCC-GB patients are different from those reported in HNSCC. Most notable is FAT1 , mutated in 28.1% ( n =110) of the OSCC-GB patients with many truncating mutations, compared with 0% (ref. 12 ) and 12% (ref. 13 ) reported earlier in HNSCC. Mutations in FAT1 promote aberrant Wnt activation that leads to tumorigenesis in various cancers [42] . FAT3 and FAT4 were also frequently mutated in OSCC-GB. FAT4 plays a crucial role in carcinogenesis as a key component of the Hippo signalling pathway and in inhibition of cell proliferation [43] . FAT3 , whose precise function is unclear, was not reported to be frequently mutated in HNSCC, but was mutated in 12% of OSCC-GB patients. We have discovered five new genes associated with OSCC-GB, one of which, USP9X , is a tumour suppressor [27] and another, MLL4 , is a co-activator of a tumour-suppressor (p53). An additional member of the MLL family, MLL2 , was also frequently mutated in 10% of OSCC-GB patients, but the estimated mutation rate in this gene was not significantly higher than the background rate. Conditional deletion of SMAD4 leads to HNSCC in the mouse [44] . SMAD4 is a central transducer of TGFβ response related tumorogenesis [45] . USP9X is a deubiquitinating enzyme for SMAD4 . Loss of USP9X therefore prevents deubiquitination of SMAD4 , enhancing tumour progression. SMG1 , frequently mutated in 12% of OSCC-GB patients, is an activity-optimizer of p53. The third new gene associated with OSCC-GB, ARID2 , is a chromatin remodelling gene, earlier reported to be frequently mutated in various cancers [46] , [47] , [48] . Some other chromatin remodelling genes ( EP300 , NSD1 , KDM5A , ARID1A, CHD7 , TET1 and HIST1H3E ) were also frequently mutated. The two remaining OSCC-GB genes discovered are UNC13C and TRPM3 , both associated with neurotransmitter processes. UNC13C is likely involved in regulating neurotransmitter release [32] . TRPM3 channels act as novel modulators of glutamatergic transmission in the developing brain [33] . The glutamatergic system appears to be critically involved in nicotine dependence [49] . It is intriguing that these genes should be somatically mutated in OSCC-GB patients, although we note that a fair proportion (26%) of patients harbour germline mutations also in UNC13C , but not in TRPM3 . TRPM3 , which is a host gene of miR-204, possibly acts synergistically with miR-204 to regulate suppression of tumour growth as well as tumour cell migration and invasion [34] . Investigations on possible functional impacts of the non-synonymous mutations found in the 10 genes that are frequently and significantly mutated in OSCC-GB, performed using bioinformatics tools PROVEAN [50] and SIFT [51] , revealed that at least 91% of the mutations are deleterious or damaging ( Supplementary Table S10 ). Three molecular subgroups of patients were identified ( Fig. 2 ). One subgroup harbours mutations in CASP8 , with mutations in FAT1 and/or NOTCH1 . The subgroup with CASP8 mutations was recognized earlier [14] . Another subgroup comprises patients with mutated TP53 , while in patients belonging to the third subgroup predominantly MLL4 and USP9X among other genes are mutated. Twelve percent of the patients harbour known oncogenic missense mutations in HRAS [52] . The HRAS mutations are known targets of therapeutic drugs of various cancers [53] . Three subsets of patients—those with CASP8 and NOTCH1 mutations with additional mutations in FAT1 (C 1.2 ) or ARID2 (C 1.4 ) and those with mutated MLL4 (C 3.2 )—comprising 16% of all patients have a significantly elevated (by 8 months) mean duration of disease-free survival compared with the pooled mean of all patients. Because of limited numbers of tumours harbouring mutations in these genes ( CASP8 , MLL4 , etc. ), the inferences on disease-free survival advantage must be accepted as preliminary, pending verification. Several new genes with CNVs were associated with OSCC-GB, some with amplifications ( DROSHA , MECOM , MMP gene cluster, YAP1 , NFIB and PSIP1 ) and others with deletions ( POLB , CCNC , DDX3X ). Somatic SNVs, but not CNVs, were identified in some of these genes in HNSCC [13] and medulloblastoma [54] . DDX3X plays an important role in apoptosis [13] . MECOM gene product functions as a transcriptional regulator binding to DNA in the promoter region of target genes and positively or negatively regulates their expression [55] . This oncogene plays an important role in development, cell proliferation and differentiation [55] . Similar to our finding, MECOM was frequently amplified in ovarian cancer [56] . The RNase III gene product of DROSHA , amplified in 12% of the OSCC-GB patients, is the core nuclease that initiates microRNA (miRNA) processing in the nucleus; alterations in the expression of Drosha are associated with cancer [57] . Nuclear factor I/B ( NFIB ), amplified in 10% of OSCC-GB patients, regulates cell viability and proliferation during transformation in the mouse squamous cell lung cancer (SCLC) model and in human SCLC [58] . Significantly high level of NFIB mRNA was found in triple negative breast cancer [59] . Other deleted genes include polymerase beta— POLB (14%), a DNA polymerase involved in base excision and repair; cyclin C— CCNC (10%), a cell cycle regulator; YWHAZ , a member of signal transduction pathway and a proto-oncogene JUN , found amplified in three OSCC-GB patients. TP63 amplification was also observed in four patients. Fibroblast growth factor receptor genes FGFR1 and FGFR4 were found altered in 10% of HPV-negative OSCC-GB tumours. These genes mediate cellular signalling. There is increasing evidence that FGFRs drive oncogenes in certain cancers and act in a cell-autonomous fashion to maintain the malignant properties of tumour cells [60] . Since autophosphorylation of one or more FGFRs is required for activation of FGF-induced downstream signalling, molecules have been developed to inhibit autophosphorylation [61] , [62] . The functional impacts of alterations in FGFR s 1 and 4 found in 10% of OSCC-GB patients require investigation in the context of the availability of inhibitor molecules for treatment. We have also identified several new pathway alterations in OSCC-GB. These include Wnt signalling, dorso-ventral axis formation and axon guidance. Recently axon guidance pathway genes were shown to be important in pancreatic cancer [30] . Integrative analysis is beginning to provide deeper insights on molecular characteristics driving OSCC [14] . In the heterogeneous class of head and neck cancers, the mutational landscape indicates that mutations in several cancer genes are specific to driving the homogeneous subset of gingivo-buccal oral squamous cell carcinoma. These specific genes are tumour suppressors or functionally associated with a known tumour suppressor, such as p53. Overall, tumour suppressor genes, compared with oncogenes, are predominantly involved in oral cancer; this fact may have therapeutic implications [14] . CNVs in genes that modulate cell cycle, apoptosis, microRNA processing, and so on, were significantly associated with gingivo-buccal oral cancer; many of these associations were not detected in earlier studies on head and neck cancer. Enrichment of alterations in new pathways was also discovered. These new findings underscore the importance of careful, high-quality investigations on homogeneous cancer subtypes using unbiased DNA sequencing. The driver mutations in the newly identified genes associated with gingivo-buccal oral cancer require functional understanding for assessment of their translational potential. Ethical approval and informed consent This study was approved by the Institutional Ethics Committees of the Advanced Centre for Treatment, Research and Education in Cancer (ACTREC), Mumbai, and the National Institute of Biomedical Genomics (NIBMG), Kalyani. All patients were recruited into this study after obtaining their voluntary informed consent. Assessment of isolated DNA and HPV infection Genomic DNA was extracted from the tumour tissue using PAXgen Tissue DNA kit (Qiagen), and from whole-blood samples using Blood DNA Mini kit (Qiagen), following the manufacturer’s protocols. The quality and DNA concentration of the samples were assessed using NanoDrop ND1000 spectrophotometer (Thermo Fisher) and 0.8% agarose gel electrophoresis. Samples with OD 260 /OD 280 ratio≥1.8, OD 260 /OD 230 ratio≥1.9, DNA concentration between 250 to 500 ng μl −1 and with no visible evidence of contamination with RNA or of DNA degradation were accepted for further genomic analysis, including exome capture and massively parallel DNA sequencing. Each tumour DNA sample was screened for the presence of HPV DNA by a PCR and DNA sequencing-based method [63] . About 100 ng of genomic DNA per sample was used for PCR with HPV L1 consensus primers (MY09 and MY11) [63] and FastStart Taq DNA Polymerase (Roche Applied Science) in ABI 9700 Gold thermal cyclers (Life Technologies) to amplify a 450-bp fragment. For each sample, 2 μl of the L1 PCR product was amplified using nested primers GP05 and GP06 targeting a 140-bp fragment. The PCR products were visualized by 2% agarose gel electrophoresis, purified by AmPure XP reagent (Beckman Coulter) and subjected to Sanger dideoxy chain termination sequencing with the PCR primers GP05 and GP06 using ABI Big Dye Terminator v3.1 sequencing kit and analysed in ABI 3500XL DNA sequencer (Life Technologies). The DNA sequences obtained were used to perform BLAST for identification of HPV types. Each tumour DNA sample was also screened for the presence of Herpes simplex virus 1 and -2 (HSV-1 and HSV-2) DNA with LightMix Kit HSV-1/2 (TIB MOL BIOL) and LightCycler FastStart DNA Master HybProbe (Roche Diagnostics). Briefly, a 214-bp fragment of HSV-1 and a 215 bp fragment of HSV-2 POL gene were amplified and detected by using hybridization probe specific for HSV-1 labelled with LightCycler Red 640 in a real-time PCR assay in LightCycler 480 instrument (Roche Diagnostics). Presence of HSV-1 and HSV-2 were discriminated by running a melting curve method after PCR, as HSV-2 amplicon–probe duplex has lower melting temperature ( T m) compared with the HSV-1 amplicon–probe duplex. False-negative PCR results were identified by an additional PCR product of 278 bp obtained from an internal control added to the reactions. Exome capture and massively parallel DNA sequencing About 62 Mb of the coding region of the human genome, comprising 201,121 exons and 9.0 Mb of miRNA coding regions, was captured using TruSeq Exome Enrichment Kit (Illumina). Briefly, for each sample, 1.5 μg of genomic DNA was used to generate fragments of size 200–300 bp by Covaris (Covaris Inc). The fragments were end-repaired by mixing with End Repair Mix (TruSeq DNA Sample Prep Kit, Illumina) and incubating at 30 °C for 30 min and purified by Ampure XP system (Beckman Coulter). These fragments were adenylated at 3′-ends with A-Tailing Mix at 37 °C for 30 min and ligated to DNA Adapter Indexes for multiplexing with DNA Ligase Mix at 30 °C for 10 min. The ligation products were purified first with Ampure XP system (Beckman Coulter) and then by 2% agarose gel eltrophoresis followed by MinElute Gel Extraction Kit (Qiagen). The DNA fragments were subsequently enriched by PCR amplification with PCR Master Mix (TruSeq DNA Sample Prep Kit, Illumina) for 10 cycles (98 °C-10 s, 60 ° for 30 s, 72 ° for 30 s) in ABI 9700 PCR system (Life Technologies) and purified with Ampure XP system (Beckman Coulter). The quality and quantity of the genomic DNA libraries thus obtained were assessed by analysing them in High Sensitivity DNA chip in 2100 Bioanalyzer (Agilent) and real-time PCR with Kapa Library Quant Kit (Kapa Biosystems) in ABI 7900HT system (Life Technologies). Genomic DNA libraries of fragment size between 300 and 400 bp and minimum yield of 500 ng were selected for exome enrichment. For exome enrichment, DNA libraries were mixed to form six-plex pools based on the sequence of index adapters used and hybridized to Capture Target Oligonucleotides (TruSeq Exome Enrichment Kit, Illumina) by incubation at 93 °C for 1 min (decreasing 2 °C per cycle for 18 cycles) followed by 58 °C for 19 h in ABI 9700 PCR system (Life Technologies). The hybridized library fragments were bound to Streptavidin Magnetic Beads and washed sequentially with Wash solutions 1, 2 and 3. These were then eluted in Elution Target Buffer 1 and 2 N NaOH and subjected to a second round of hybridization to Capture Target Oligonucleotides (TruSeq Exome Enrichment Kit, Illumina) and elution as above. The eluted exome-enriched library fragments were PCR-amplified for 12 cycles (98 °C for 10 s, 60 °C for 30 s, 72 °C for 30 s) in ABI 9700 PCR system (Life Technologies) and purified with Ampure XP system (Beckman Coulter). The enriched DNA libraries were quantified by real time PCR with Kapa Library Quant Kit (Kapa Biosystems) in ABI 7900HT system (Life Technologies). Each exome-enriched 6-plex DNA library pool was paired-end-sequenced for 210 cycles in at least two lanes of HiSeq-2000 System (Illumina) using TruSeq PE Cluster Kit v3 and TruSeq SBS Kit v3 (Illumina). In a concurrent orthogonal approach, ~26 Mb of the coding region of the human genome, comprising 180,000 coding exons from the CCDS database and 551 miRNA coding regions, was captured with 2.1 million probes in the Seq Cap EZ Exome Capture Probe Library (Roche-NimbleGen). For each sample, genomic DNA fragments of size range 500–800 bp were generated by nebulization of 1 μg of purified genomic DNA with nitrogen gas at 30 psi pressure for 1 min. The nebulized DNA was purified by MinElute PCR Purification kit (Qiagen), end polished with T4 DNA Polymerase, Polynucleotide Kinase and Taq DNA Polymerase (Roche) by incubation at 25 °C for 20 min and 72 °C for 20 min followed by ligation of library adapter oligonucleotides using DNA Ligase (Roche). The genomic DNA libraries were then purified by Ampure XP (Beckman Coulter). These genomic DNA libraries were then PCR-amplified in 10 cycles (95 °C for 30 s, 64 °C for 30 s, 72 °C for 3 min) with FastStart High Fidelity Enzyme Blend (Roche) and Rapid-A and Rapid-B oligonucleotides (Roche-NimbleGen Rapid Library kit) in ABI 9700 PCR system (Life Technologies). The PCR products were purified by QIAquick PCR Purification kit (Qiagen) and hybridized to Seq Cap EZ exome capture probes (Roche-NimbleGen) along with COT DNA and Rapid HE1 and HE2 oligonucleotides at 47 °C for 70 h. The hybridized DNA fragments were then bound to streptavidin-Dynabeads (Invitrogen) at 47 °C for 45 min, washed and directly amplified from bound Dynabeads by 15 cycles of PCR as mentioned above. The amplified products were purified by QIAquick PCR Purification kit (Qiagen). The quality of the exome libraries obtained were assessed by analysing them using DNA 7500 chip in 2100 Bioanalyzer (Agilent) and quantified using Picogreen dye in Qubit Fluorometer (Invitrogen). The extent of exome enrichment in the DNA libraries was assessed by SYBR-Green Real Time PCR based relative quantitation of four exon targets of genes RUNX2 , PRKG1 , SMG1 and NLK . Libraries with fragment size between 500 and 800 bp, of minimum quantity 1 μg and minimum enrichment of 100-fold in at least three out of the 4 exon targets in Real Time PCR were selected for deep sequencing. Each blood and tumour exome library was then sequenced at minimum depth of 25 × and 40 × respectively using Titanium series chemistry (Roche). Briefly, for each sequencing run, 2 × 10 7 exome library molecules were clonally amplified by emulsion PCR in ABI 9700 PCR systems (Life Technologies), purified using REMe integration (Roche) on Biomek 3000 (Beckman Coulter) and pyrosequenced in pico-titre plates in GS-FLX Genome Sequencers (Roche) and Titanium chemistry (Roche). Initial analyses of massively parallel DNA sequence data The exome-sequencing data generated on HiSeq 2000 were analysed using FASTQC [64] for quality checking. BWA [65] was used for alignment and mapping of reads against hg19 with decoy sequences as used in 1,000 Genomes project [66] . SAMtools [67] was used for conversion of SAM files to BAM files and for pile up after local alignment. Specific modules of GATK [68] were used for local alignment around insertions/deletions and base-quality score recalibration. Details of initial analysis of Gs-FLX (454) data are provided in Supplementary Methods. Statistical inferences on nature of genomic alteration Initial standard statistical methods of analysis are presented in Supplementary Methods . Here we describe a new statistical method for variant calling implemented in the base-by-base (BbB) variant caller ( Supplementary Methods ) developed by us and used here. Let n denote the total number of reads covering a locus (site), n 1 the number of reads with the reference allele (R), and n − n 1 the number of reads with the variant allele (V). Let π denote the probability that the allele is R, in blood. The null hypotheses of interest are: (i) π =1 (if n 1 ≥ n − n 1 ) or (ii) π =0 (if n 1 < n − n 1 ). We note that if π =1 (or 0), then n 1 (or n 2 ) must equal n . However, in practice this does not happen, because of errors on massively parallel sequencing platforms. For example, even if the genotype at the locus is RR, there are some variant reads. Let the ‘machine error rate’ as denoted as ε (numerically small, ~0). In view of the above, instead of testing the null hypotheses (i) and (ii), we test: (i′) π =1−ε (if n 1 ≥ n - n 1 ) or (ii′) π =0+ε (if n 1 < n − n 1 ). If the null hypothesis (i′) is accepted, then the genotype in blood is RR; if (ii′) is accepted, then the genotype is VV; and, if neither hypothesis is accepted, then the genotype is RV. Unless, ultra-deep sequencing is performed, the total number of reads ( n ) is often small. This may lead to the rejection of both hypotheses and therefore by default to making a heterozygote call when in fact there may not be sufficient strength of statistical evidence favoring a heterozygote call (because of the small number of reads). To avoid vagaries of making spurious calls ‘by default’, when both hypotheses were rejected, we further tested the null hypothesis (iii) π =0.5−ε (or, 0.5+ε). There were instances, when both (i′) and (ii′) were rejected and (iii) was also rejected (or, (i′) or (ii′) were accepted and (iii) was also accepted); in such instances, we did not make a call at that locus and scored it as ‘missing genotype’, thereby avoiding incorrect scoring of genotypes. A binomial test of proportions was carried out to test each of the null hypotheses stated above. P -values were calculated by evaluating the probability that a binomial random variable ( n , π) assumes a value greater than the observed number of reference (or variant) reads, n 1 (or n − n 1 ). We used Benjamini−Hochberg False Discovery Rate of 0.01 to reject a null hypothesis. We empirically estimated the value of the ‘machine error rate’, ε . Essentially, since in each sequencing run data on some ‘control sequences’ are automatically generated, these data were used to estimate ε . Estimates of ε varied between 0.0015 and 0.013, across sequencers and runs ( Supplementary Fig. S5 ). We have used ε =0.01 (a conservative upper limit) in all our calculations. Using statistical methodology similar to that described above, data on tumour DNA were also analysed. The overview of the methodology and inferences is depicted in Supplementary Fig. S6 and Supplementary Table S11 . Verification of somatic mutations Variant sites of acceptable quality that were present in HiSeq 2000 data, but were outside of the Nimblegen capture region and hence not present in GS-FLX data, and frequently mutated in ≥10% of the patients, were verified using the Ion Torrent platform. Sanger sequencing was done for TP53. Details are provided in Supplementary Methods . Genome-wide SNP scan and CNV detection Each DNA sample was genotyped for 1.14 million SNP markers using Illumina Omni Quad arrays and scanned on iScan (Illumina). The results were analysed by Genome Studio Illumina Genome Studio v2011.1 (genotyping module 1.4.9). CNV detection from these data was performed using ASCAT [69] . Details are provided in Supplementary Methods . Real-time PCR assays were performed ( Supplementary Methods , Supplementary Table S12 ) for representative somatic CNVs for confirmation of ASCAT results. Identification of SMGs We identified genes that are significantly mutated by statistically comparing the observed numbers of mutations to the numbers expected to accumulate if the genes were evolving at background mutation rate (BMR). These calculations were carried out using Genome MuSiC package, Ver. 0.4 (ref. 23 ). This algorithm appropriately adjusts mutation rates for gene-length and base-composition. We have used the number of nucleotides in the coding segment of a gene as the length of the gene. Only the number of bases with adequate coverage in both blood and tumour BAM files for each patient was used. For each gene, to test the significance of enhanced mutations compared with the background rate, MuSiC calculates three test-statistics—Fisher’s combined P -value test (FCPT), Likelihood-Ratio test (LRT) and the Convolution test (CT)—and then estimates the P -value and the false discovery rate (FDR). In this study, a gene with FDR<0.2 in at least two of the three tests and also recurrently mutated in at least 10% of the patients was declared as a SMG. We have also applied the MutSigCV v1.3 algorithm [24] for an independent validation of SMGs. MutSigCV estimates the background mutation rate for each gene–patient–category set based on the observed silent mutations in the gene and non-coding mutations in the neighbouring regions. MutSigCV uses patient-specific mutation frequency and spectrum, and gene-specific background mutation rates incorporating expression level and replication time to identify SMGs. The null hypothesis that the observed number of mutations in a gene is equal to that expected under the background mutation rate is tested using standard statistical methods. Nucleotide context To understand the mutational processes that drive the C>X (X being any one of the four nucleotides) mutations, we identified nucleotides flanked immediately 5′ and 3′ of the mutated cytosine bases from the human genome reference sequence (hg19) from both strands. Expected distribution of 5′X-C-3′X sequence motif in exons of the human genome (hg19) was obtained by random sampling of 10,000 cytosine bases. For each sampled cytosine base, the 16 possible 5′X-C-3′X nucleotide contexts were noted, and their frequencies determined. These served as expected frequencies. Frequencies of the various nucleotide contexts in which C>X mutations were observed among OSCC-GB patients were statistically compared with the expected frequencies using a 2 × 16 contingency χ 2 test. If the χ 2 test was significant, then we statistically tested (using Z -test of equality of proportions) whether frequencies of specific 5′X-C-3′X context categories were enriched in OSCC-GB patients compared with those expected. Pathway analysis PathScan module in GenomeMuSiC package [23] was used to discover significant pathways enriched with somatic mutations in annotated KEGG (Kyoto Encyclopedia of Genes and Genomes) pathways. PathScan uses the two features in the pathway analysis: variation in gene lengths and the consequent differences of their mutation likelihood under the null hypothesis, and distributions of mutations among samples and their combination into an overall P -value. We have used only the coding segment of a gene as its length in PathScan calculations. All pathways comprising <10 genes (16 such pathways) from the KEGG database were removed. One hundred and ninety KEGG pathways were subsequently used as the input pathway database in GenomeMuSiC package. Only those non-silent somatic variations that, as per UniProt annotation, affect active domains of a protein were used as inputs for pathway analysis in PathScan module. Significantly overrepresented gene pathways in gingivo-buccal oral cancer ( P <0.05) were used for our further analysis. Non-relevant pathways such as olfactory transduction pathways were removed from the final report. Accession codes: Sequence BAM files have been deposited in the European Genome-Phenome Archive under accession code EGAS00001000249. How to cite this article: India Project Team of ICGC. Mutational landscape of gingivo-buccal oral squamous cell carcinoma reveals new recurrently-mutated genes and molecular subgroups. Nat. Commun. 4:2873 doi: 10.1038/ncomms3837 (2013).